Non-transgenic genome modifications in a hemimetabolous insect using zinc-finger and TAL effector nucleases Hemimetabolous, or incompletely metamorphosing, insects are phylogenetically relatively basal and comprise many pests. However, the absence of a sophisticated genetic model system, or targeted gene-manipulation system, has limited research on hemimetabolous species. Here we use zinc-finger nuclease and transcription activator-like effector nuclease technologies to produce genetic knockouts in the hemimetabolous insect Gryllus bimaculatus . Following the microinjection of mRNAs encoding zinc-finger nucleases or transcription activator-like effector nucleases into cricket embryos, targeting of a transgene or endogenous gene results in sequence-specific mutations. Up to 48% of founder animals transmit disrupted gene alleles after zinc-finger nucleases microinjection compared with 17% after microinjection of transcription activator-like effector nucleases. Heterozygous offspring is selected using mutation detection assays that use a Surveyor (Cel-I) nuclease, and subsequent sibling crosses create homozygous knockout crickets. This approach is independent from a mutant phenotype or the genetic tractability of the organism of interest and can potentially be applied to manage insect pests using a non-transgenic strategy. Continuous improvements in DNA sequencing technologies continue to facilitate sequence analyses of complete genomes of numerous species. Moreover, the ability to directly and specifically manipulate a genome, for example, by generating specific gene knockouts, is essential for elucidating gene function on a genome-wide scale. However, the molecular tools and methods needed for gene targeting require a functional genomics approach. Thus, these techniques have been limited to the study of certain well-established model organisms, including yeast [1] , fruitflies [2] and mice [3] , although approaches in these systems are still often inefficient. As a result, a systematic, reverse genetic analysis of crickets, and perhaps other lesser-studied species, has been limited by the absence of a suitable genome-manipulation technique, until now. Engineered nucleases, including zinc-finger nucleases (ZFNs) and transcription activator-like effector nucleases (TALENs), are powerful tools for genome editing based on their capacity to target a specific genomic locus [4] , [5] . For example, ZFNs can be generated by linking the nonspecific cleavage domain of the Fok I restriction endonuclease to a DNA-binding domain composed of modular zinc-finger (ZF) domains [4] . Each ZF domain primarily contacts three base pairs (bps) within the major groove of DNA. However, ZFs can be modified to recognize a broad range of DNA sequences [4] , [6] . Ideally, a pair of ZFNs is designed for a particular target, whereby dimerization of the associated cleavage domains is accommodated and a double-stranded break (DSB) is introduced ( Fig. 1a ) [6] , [7] . Alternatively, TALENs consist of an engineered array of TAL effector repeats fused to the Fok I cleavage domain, and can also introduce targeted DSBs in DNA [5] . The DNA-binding domains of TALEs have tandem repeat units (each 33–35 aa in length), in which the nucleotide binding preference is determined by the two adjacent amino acids, and these are referred to as the repeat variable di-residue [8] . For both systems, DSBs can be restored via cellular DNA repair pathways, which include non-homologous end-joining (NHEJ) mechanisms and homologous recombination mechanisms. For NHEJ-based repairs of ZFN/TALEN-induced DSBs, small insertions and/or deletions (indels) are produced at the repair junction, thereby generating mutations precisely at the cleavage site ( Fig. 1a ) [9] . 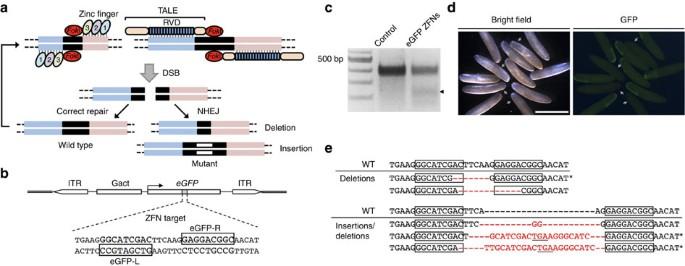Figure 1: Disruption of aneGFPtransgene inG. bimaculatususing designed ZFNs. (a) Illustration of the binding and function of ZFNs and TALENs. Following the introduction of double-stranded breaks (DSB) in the DNA between targeted binding sites, these breaks are either repaired and digested again, or NHEJ can occur and deletions or insertions can result. In the latter case, gene function of the targeted gene is disrupted, and subsequent binding of ZFNs or TALENs does not result inFokI dimerization or the generation of DSBs. (b) Structure of the pBGact-eGFPtransgene that is under the transcriptional control of theGrylluscytoplasmicactinpromoter (Gact) and flanked by 5′ and 3′ inverted terminal repeats (ITRs). The 9-bp binding sites for the ZFNs, eGFP-R and eGFP-L are in the boxes shown. (c) Detection of induced mutations into genomic DNA cleaved by Surveyor nuclease that was collected from embryos injected with both eGFP-R and eGFP-L mRNAs or eGFP-R mRNA alone (control) at 7 days postinjection. A product cleaved by Surveyor nuclease was detected in the genomic DNA from embryos injected with eGFP-R/L mRNAs (arrowhead). (d) Bright field (left panel) and fluorescence (right panel) phenotypes of G1crickets injected witheGFPZFN mRNA at 2 days after egg laying. While the embryos appeared to develop normally, some embryos did not exhibiteGFPfluorescence (indicated with arrows). Scale bar, 2.5 mm. (e) Sequence analysis ofeGFPmutant alleles induced byeGFPZFN mRNAs. Wild-type (WT) sequences are shown above the mutant sequences containing deletions (indicated with dashes) and/or insertions (shown in red letters). Asterisks indicate knockout mutations that included frame-shift and stop codon insertions (underlined). Figure 1: Disruption of an eGFP transgene in G. bimaculatus using designed ZFNs. ( a ) Illustration of the binding and function of ZFNs and TALENs. Following the introduction of double-stranded breaks (DSB) in the DNA between targeted binding sites, these breaks are either repaired and digested again, or NHEJ can occur and deletions or insertions can result. In the latter case, gene function of the targeted gene is disrupted, and subsequent binding of ZFNs or TALENs does not result in Fok I dimerization or the generation of DSBs. ( b ) Structure of the pBGact- eGFP transgene that is under the transcriptional control of the Gryllus cytoplasmic actin promoter (Gact) and flanked by 5′ and 3′ inverted terminal repeats (ITRs). The 9-bp binding sites for the ZFNs, eGFP-R and eGFP-L are in the boxes shown. ( c ) Detection of induced mutations into genomic DNA cleaved by Surveyor nuclease that was collected from embryos injected with both eGFP-R and eGFP-L mRNAs or eGFP-R mRNA alone (control) at 7 days postinjection. A product cleaved by Surveyor nuclease was detected in the genomic DNA from embryos injected with eGFP-R/L mRNAs (arrowhead). ( d ) Bright field (left panel) and fluorescence (right panel) phenotypes of G 1 crickets injected with eGFP ZFN mRNA at 2 days after egg laying. While the embryos appeared to develop normally, some embryos did not exhibit eGFP fluorescence (indicated with arrows). Scale bar, 2.5 mm. ( e ) Sequence analysis of eGFP mutant alleles induced by eGFP ZFN mRNAs. Wild-type (WT) sequences are shown above the mutant sequences containing deletions (indicated with dashes) and/or insertions (shown in red letters). Asterisks indicate knockout mutations that included frame-shift and stop codon insertions (underlined). Full size image ZFN-targeted mutations have been induced in several organisms, including fruitflies [10] , [11] , [12] , silkworms [13] , zebrafish [14] , rats [15] , [16] , sea urchins [17] , roundworms [18] , frogs [19] and mice [20] , [21] . More recently, TALENs have been applied to rats [22] , zebrafish [23] and fruitflies [24] . In both models, mRNA was directly injected into embryos. However, the success of this method in engineering homozygous knockout animals that exhibit null phenotypes has had limited success, and has only been reported in fruitflies [10] , [24] , zebrafish [14] , [23] and rats [15] , [16] , [22] . In these cases, selective breeding with animals that bear specific genetic markers, or morphologically detectable phenotypes, was performed after ZFN mutagenesis. Correspondingly, these approaches depended on genetic tractability, or the characteristics of the phenotypes generated. To facilitate a more generally applicable knockout analysis in various organisms, including non-model ones, a strategy to apply ZFN/TALEN-mediated mutagenesis for the generation of homozygous knockout animals was investigated. The cricket, Gryllus bimaculatus (Orthoptera), is an emerging model system that has been used to study developmental biology and mechanisms of regeneration based on the success of RNA interference (RNAi)-based gene-functional analyses and transgenic technology in this system [25] , [26] . It is possible that this cricket model could also be used to characterize the molecular mechanisms relevant to human diseases, and be a model for the screening of therapeutic drugs with RNAi [27] . However, while the cricket is currently used as a model system in the fields of neuroethology, endocrinology and behavioural ecology, the introduction of targeted and heritable mutations has remained intractable in this species. Therefore, the ability to edit the cricket genome would further enhance studies performed in all of these fields. Here we report the generation of homozygous knockouts of an endogenous gene in G. bimaculatus via ZFN- and TALEN-based targeted mutagenesis. A simple, efficient and broadly applicable approach is described for the construction of gene knockouts, and this approach involves the direct injection of mRNAs encoding ZFNs or TALENs into embryos, combined with mutant detection assays that use the Surveyor (Cel-I) nuclease. Testing the functionality of ZFNs in cricket embryos As proof of principle, the function of ZFNs targeted to an eGFP ( enhanced green fluorescent protein ) transgene in the cricket genome was evaluated. Specifically, two ZFNs, eGFP-L and eGFP-R, were designed to target the coding region of the eGFP gene ( Fig. 1b ; Table 1 ). To generate these functional ZFNs, a bacterial one-hybrid (B1H) system using randomized libraries of ZF domains and single-strand annealing (SSA) assays performed in cultured cells were used [17] , [28] . The ZF proteins assembled were linked to variants of the Fok I nuclease domain. These variants functioned as obligate heterodimers to reduce their propensity for homodimerization, thereby decreasing the frequency of off-target cleavage events [29] . Coinjections of mRNAs of eGFP-L and eGFP-R into heterozygous eGFP transgenic cricket eggs were then performed [26] . As negative controls, eGFP-L or eGFP-R mRNAs were injected individually. After 7 days, genomic DNA was extracted from ZFN-treated and control embryos in the G 0 generation, and the mismatch-sensitive endonuclease, Surveyor (Cel-I) [30] , was used to screen these DNA samples. The results of these assays demonstrated that mutations were induced in the targeted locus of ZFN-treated embryos, yet not in the controls ( Fig. 1c ). Moreover, fluorescence was detected in the G 1 generation of transgenic cricket embryos carrying eGFP in the control group (untreated), and not in a subset of ZFN-treated embryos ( Fig. 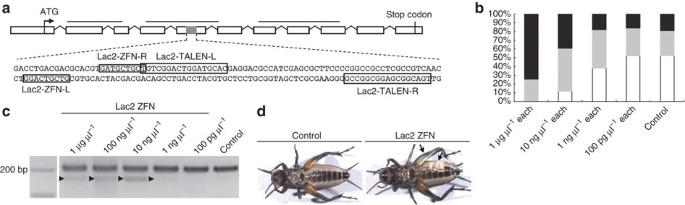Figure 2: Design and application of ZFNs and TALENs targeted toGb′lac2. (a) Structure of theGb′lac2gene, with open boxes representing exons mapped on theGryllusgenomic sequence. Black bars indicate Cu-oxidase domains 1–3. The grey region of the fifth exon is expanded to provide the gene sequence that includes the 9 or 17 bp ZFN and TALEN binding sites, respectively (shown in boxes). (b) Dose-dependent toxicity ofGb′lac2ZFN mRNAs in cricket embryos. The percentages of dead (black), deformed (grey) and normal (white) embryos at 2 days postinjection are shown. The control was embryos injected with Lac2-L ZFN mRNA alone. The percentage of embryos that developed normally increased with decreasing concentrations ofGb′lac2ZFN mRNAs (0/43 for 1 μg μl−1each, 6/51 for 10 ng μl−1each, 19/50 for 1 ng μl−1each, 13/25 for 100 pg μl−1each and 11/21 for control). (c) Using a Surveyor nuclease assay, mutations inGb′lac2were detected following the microinjection of crickets withGb′lac2ZFN mRNAs. Products cleaved by Surveyor nuclease (indicated with arrowheads) were detected at 1 μg μl−1, 100 ng μl−1, 10 ng μl−1and 1 ng μl−1of Lac2 ZFN injected. (d) Imaging of control andGb′lac2ZFN final-instar nymphs. Mutagenesis of somatic cells in G0crickets was detected based on the presence of a white spot phenotype by epidermal cells (indicated with arrows). 1d ; Table 2 ). Subsequent sequence analyses of targeted loci in the G 1 embryos revealed that the ZFN-induced mutations contained multiple indels ranging from 4 to 28 bp centred over the ZFN recognition site ( Fig. 1e ). These results indicate that the mutations present resulted from NHEJ. Thus, a lack of eGFP -encoded fluorescence and mutations of the wild-type eGFP DNA sequence indicated that knockout of the eGFP transgene had been achieved. In combination, these results show that engineered ZFNs can induce mutations in a targeted locus of the cricket genome, and this DSB induces error-prone NHEJ repair. Table 1 eGFP and Gb ′ lac2 ZFNs target sites and amino-acid sequences of designed ZF recognition helices. Full size table Table 2 ZFN- or TALEN-induced mutagenesis after mRNA microinjection in insects. Full size table Mutagenesis of an endogenous gene with ZFNs To evaluate the capacity for a ZFN to produce a knockout model, disruption of the endogenous phenoloxidase gene G. bimaculatus laccase2 ( Gb ′ lac2 ) was targeted. This gene was selected based on previous studies in which RNAi targeting of Gb ′ lac2 in the nymphal stages of the cricket resulted in loss of cuticle tanning after molting [25] . An open reading frame sequence appropriate for the assembly of ZFNs was identified in the second oxidase domains of the Gb ′ lac2 gene ( Fig. 2a ; Table 1 ). To achieve a high efficiency of mutagenesis, derivatives of the Sharkey cleavage domain were used for the assembly of ZFNs [31] . The mRNA of assembled ZFNs was then injected into cricket eggs. After 2 days, morphological defects were observed. All embryos injected with 1 μg μl −1 Gb ′ lac2 ZFN mRNA died, or exhibited abnormal development ( Fig. 2b ). Furthermore, when ZFN mRNAs were administered at lower concentrations, abnormal development was reduced, and 2 days after injection, embryos were comparable to normal control embryos (for example, embryos only injected with Lac2-L; Fig. 2b ). The Surveyor nuclease assay was able to detect the ZFN-induced mutations in embryos injected with each Gb ′ lac2 ZFN mRNA at the reduced concentration of 1 ng μl −1 , at least ( Fig. 2c ). Hatched nymphs were also reared from embryos injected with 1 ng μl −1 mRNAs, and ~58% of the fifth-instar G 0 larvae of this group exhibited a mosaic cuticle pattern with and without tanning ( Fig. 2d ; Table 2 ). Therefore, the presence of somatic mutants was confirmed. Figure 2: Design and application of ZFNs and TALENs targeted to Gb′lac2 . ( a ) Structure of the Gb ′ lac2 gene, with open boxes representing exons mapped on the Gryllus genomic sequence. Black bars indicate Cu-oxidase domains 1–3. The grey region of the fifth exon is expanded to provide the gene sequence that includes the 9 or 17 bp ZFN and TALEN binding sites, respectively (shown in boxes). ( b ) Dose-dependent toxicity of Gb ′ lac2 ZFN mRNAs in cricket embryos. The percentages of dead (black), deformed (grey) and normal (white) embryos at 2 days postinjection are shown. The control was embryos injected with Lac2-L ZFN mRNA alone. The percentage of embryos that developed normally increased with decreasing concentrations of Gb ′ lac2 ZFN mRNAs (0/43 for 1 μg μl −1 each, 6/51 for 10 ng μl −1 each, 19/50 for 1 ng μl −1 each, 13/25 for 100 pg μl −1 each and 11/21 for control). ( c ) Using a Surveyor nuclease assay, mutations in Gb ′ lac2 were detected following the microinjection of crickets with Gb ′ lac2 ZFN mRNAs. Products cleaved by Surveyor nuclease (indicated with arrowheads) were detected at 1 μg μl −1 , 100 ng μl −1 , 10 ng μl −1 and 1 ng μl −1 of Lac2 ZFN injected. ( d ) Imaging of control and Gb ′ lac2 ZFN final-instar nymphs. Mutagenesis of somatic cells in G 0 crickets was detected based on the presence of a white spot phenotype by epidermal cells (indicated with arrows). Full size image Generation of homozygous knockout crickets To generate a homozygous knockout of Gb ′ lac2 , a simple genetic scheme was designed where mates with a specialized genetic background were not needed ( Fig. 3a ). As the first step, ZFN-treated G 0 crickets (with and without somatic mutations) were crossed with wild-type crickets. Genomic DNA was then extracted from a batch of embryos derived from each cross, and Surveyor nuclease-based assays were performed to detect germline-transmitted mutations (first-round screening; Fig. 3b ). Founder crickets transmitting mutations were detected in ~47% of G 0 adults ( Table 2 ). Embryos from the Surveyor-positive lines were then collected, hatched into nymphs, and reared. Genomic DNA was extracted from the T3 leg of 16 individual final-instar nymphs from each of the four positive lines identified in the first-round screening, and Surveyor nuclease-based assays were performed (second-round screening), followed by DNA sequencing ( Fig. 3c,d ). Surveyor-positive nymphs were obtained at a rate of 31–68% for each line, and these were reared to obtain G 1 adult crickets containing heterozygous mutant alleles. Sequencing of the ZFN-targeted locus in these mutants revealed that first round–positive lines often contained multiple mutant alleles ( Fig. 3e ). 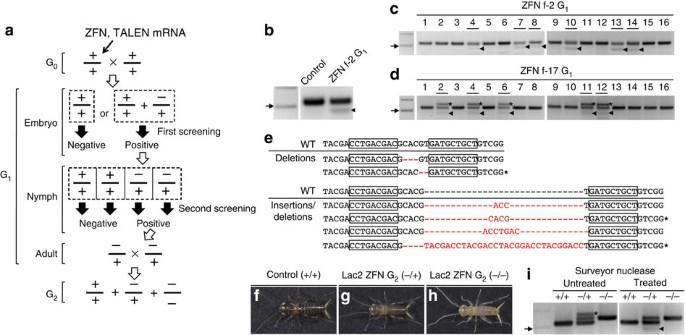Figure 3: Isolation of homozygous mutants after injection ofGb′lac2ZFN mRNAs into crickets. (a) An illustration of the scheme used to isolate homozygous mutations in an endogenous gene. Mutagenized G0adults were crossed to wild-type (WT) adults, and G1embryos were checked for heterozygous mutations in a first round of screening using the Surveyor nuclease. Positive G1individuals were developed into final-instar nymphs and subjected to a second round of screening with Surveyor nuclease assays. Positive G1adults were then crossed for each strain to obtain homozygous mutants in G2generation. (b) Germline mutations in G0crickets were detected in a first-round screening of G1embryos using Surveyor nuclease assays. The arrowhead indicates the product cleaved by the Surveyor nuclease in the f-2 line. Arrow indicates 200-bp size marker. (c,d) Isolation of heterozygous mutants from G1crickets in f-2 (c) and f-17 (d) lines detected in the second round of screening. Heterozygous mutant G1crickets were detected in a second round of screening of T3 legs from G1final-instar nymphs. Nymphs that harboured mutations caused by ZFNs are underlined. Arrowheads indicate the products generated from Surveyor nuclease assays. Asterisks indicate the presence of homoduplex PCR products from mutant alleles. Arrows indicate 200-bp size marker. (e) Sequence analysis ofGb′lac2mutant alleles induced by ZFNs. Wild-type sequences are shown above the mutant sequences containing deletions (indicated with dashes) and/or insertions (shown in red letters). Boxed sequences represent ZFN-binding sites. Asterisks indicate frame-shift mutations are present. (f–h) Phenotypes of G2heterozygous and homozygous mutant crickets 1 day after hatching. Control first-instar nymphs were coloured black until 1 day posthatching, while heterozygous mutants were still grey in colour and homozygous mutants were white. (i) Genotyping of G2heterozygous and homozygous mutants. In Surveyor nuclease assays, cleavage products were detected in heterozygous mutants (indicated with an arrowhead), but not in WT or homozygous mutants (right panel). The asterisk indicates heteroduplex PCR products from WT and mutant alleles were present. Arrow indicates 200-bp size marker. Figure 3: Isolation of homozygous mutants after injection of Gb′lac2 ZFN mRNAs into crickets. ( a ) An illustration of the scheme used to isolate homozygous mutations in an endogenous gene. Mutagenized G 0 adults were crossed to wild-type (WT) adults, and G 1 embryos were checked for heterozygous mutations in a first round of screening using the Surveyor nuclease. Positive G 1 individuals were developed into final-instar nymphs and subjected to a second round of screening with Surveyor nuclease assays. Positive G 1 adults were then crossed for each strain to obtain homozygous mutants in G 2 generation. ( b ) Germline mutations in G 0 crickets were detected in a first-round screening of G 1 embryos using Surveyor nuclease assays. The arrowhead indicates the product cleaved by the Surveyor nuclease in the f-2 line. Arrow indicates 200-bp size marker. ( c , d ) Isolation of heterozygous mutants from G 1 crickets in f-2 ( c ) and f-17 ( d ) lines detected in the second round of screening. Heterozygous mutant G 1 crickets were detected in a second round of screening of T3 legs from G 1 final-instar nymphs. Nymphs that harboured mutations caused by ZFNs are underlined. Arrowheads indicate the products generated from Surveyor nuclease assays. Asterisks indicate the presence of homoduplex PCR products from mutant alleles. Arrows indicate 200-bp size marker. ( e ) Sequence analysis of Gb ′ lac2 mutant alleles induced by ZFNs. Wild-type sequences are shown above the mutant sequences containing deletions (indicated with dashes) and/or insertions (shown in red letters). Boxed sequences represent ZFN-binding sites. Asterisks indicate frame-shift mutations are present. ( f – h ) Phenotypes of G 2 heterozygous and homozygous mutant crickets 1 day after hatching. Control first-instar nymphs were coloured black until 1 day posthatching, while heterozygous mutants were still grey in colour and homozygous mutants were white. ( i ) Genotyping of G 2 heterozygous and homozygous mutants. In Surveyor nuclease assays, cleavage products were detected in heterozygous mutants (indicated with an arrowhead), but not in WT or homozygous mutants (right panel). The asterisk indicates heteroduplex PCR products from WT and mutant alleles were present. Arrow indicates 200-bp size marker. Full size image To produce homozygous mutants, G 1 mutant siblings with identical mutations were mated. From these crosses, ~43% of hatched G 2 nymphs exhibited a lag in tanning ( Fig. 3f,g ), while 19% failed to tan ( Fig. 3h ). In the latter case, it appeared that a homozygous knockout of the Gb ′ lac2 gene had been achieved. Homozygosity was confirmed with Surveyor nuclease-based genotyping ( Fig. 3i ) and sequencing. However, homozygous knockout crickets died in the first-instar stage. To examine whether the ZFNs that were introduced caused off-target mutations, we performed a computational scan of a preliminary draft assembly of the G. bimaculatus genome (T.M. et al ., unpublished data). On the basis of nine sites identified as the most likely to represent off-target sites of ZFN cleavage ( Table 3 ), assays of these nine loci in heterozygous (G 1 ) mutant genomes were performed independently for three mutant lines using Surveyor nuclease assays. No cleavage products were detected. Assuming that the efficiency of PCR amplification is equivalent between mutated and wild-type sequences at each of the loci, the Surveyor nuclease assay would be predicted to be able to detect mutations with an equivalent sensitivity as demonstrated with the Gb ′ lac2 locus. If so, then our results indicate that unwanted mutations did not occur at the targeted genomic sites in these experiments. Furthermore, sequencing of potential off-target sites in the Gb ′ lac2 mutant genomes supported the data obtained from Surveyor nuclease assays. Table 3 Analysis of potential off-target sites of Gb ′ lac2 ZFNs. Full size table Gene knockout using TALENs The gene knockout strategy developed for ZFNs proved to be robustly applicable to TALENs. To disrupt the Gb ′ lac2 gene, a pair of TALENs targeted to the Gb ′ lac2 locus was designed (Lac2-TALEN-L and Lac2-TALEN-R; Fig. 2a ). These TALEN mRNAs were then injected into cricket eggs. In contrast with the toxicity associated with Gb ′ lac2 ZFN mRNAs, the Gb ′ lac2 TALEN mRNAs did not induce significant toxicity at 1 μg μl −1 compared with embryos injected with Lac2-L alone ( Fig. 4a ). Thus, 1 μg μl −1 was adopted as the concentration used for subsequent TALEN experiments. Of the fifth-instar G 0 larvae generated, ~17% represented somatic mutants with a mosaic cuticle pattern with and without tanning ( Table 2 ). Furthermore, the results of Surveyor nuclease-based assays with G 1 embryos (first-round screening; Fig. 3a ) suggested that mutations were induced in the targeted locus ( Fig. 4b ), and founder crickets represented ~17% of G 0 adults ( Table 2 ). Following a screening of heterozygous mutants in G 1 nymphs (second-round screening; Figs. 3a and 4c,d ) and mating of G 1 mutant siblings, homozygous Gb ′ lac2 knockout crickets were obtained ( Fig. 4e–g ). Sequencing of the TALEN-targeted locus in these mutants revealed the presence of indels, which is consistent with the induction of error-prone NHEJ repair after introduction of a DSB ( Fig. 4h ). 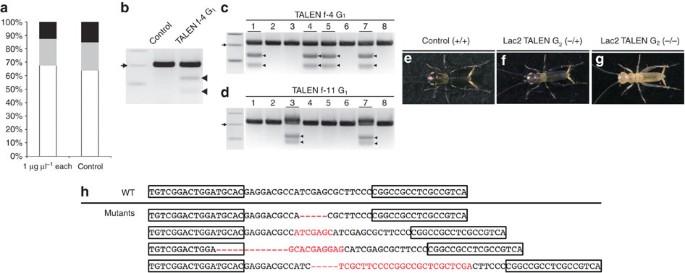Figure 4: Isolation of homozygous mutants induced by the microinjection ofGb′lac2TALEN mRNA into crickets. (a) Toxicity ofGb′lac2TALEN mRNAs in cricket embryos was detected. Percentages of dead (black), deformed (grey) and normal (white) embryos are shown at 2 days postinjection. The control included embryos injected with Lac2-L TALEN mRNA alone. The percentage of embryos that developed normally after microinjection ofGb′lac2TALEN mRNAs (68%, 82/121) was comparable to control (64%, 30/47). (b) Germline mutations in G0crickets were detected in a first-round screening of G1embryos. Arrowheads indicate the cleavage products generated in Surveyor nuclease assays of the f-4 line. Arrow indicates 200-bp size marker. (c,d) A second round of Surveyor nuclease assays was performed to identify heterozygous mutants present in G1crickets from the f-4 (c) and f-11 (d) lines. Adults that harboured mutations caused by TALENs are underlined, while arrowheads indicate cleavage products from Surveyor nuclease assays. Arrows indicate 200-bp size marker. (e–g) Phenotypes of G2heterozygous and homozygousGb′lac2mutants generated with TALENs 1 day after hatching. Control first-instar nymphs were coloured black, while heterozygous mutants were still grey in colour and homozygous mutants were white. (h) Sequence analysis ofGb′lac2mutant alleles induced by TALENs. The wild-type (WT) sequence is shown above the mutant sequences containing deletions (indicated with dashes) and/or insertions (shown in red letters). Boxed sequences represent TALEN-binding sites. Figure 4: Isolation of homozygous mutants induced by the microinjection of Gb′lac2 TALEN mRNA into crickets. ( a ) Toxicity of Gb ′ lac2 TALEN mRNAs in cricket embryos was detected. Percentages of dead (black), deformed (grey) and normal (white) embryos are shown at 2 days postinjection. The control included embryos injected with Lac2-L TALEN mRNA alone. The percentage of embryos that developed normally after microinjection of Gb ′ lac2 TALEN mRNAs (68%, 82/121) was comparable to control (64%, 30/47). ( b ) Germline mutations in G 0 crickets were detected in a first-round screening of G 1 embryos. Arrowheads indicate the cleavage products generated in Surveyor nuclease assays of the f-4 line. Arrow indicates 200-bp size marker. ( c , d ) A second round of Surveyor nuclease assays was performed to identify heterozygous mutants present in G 1 crickets from the f-4 ( c ) and f-11 ( d ) lines. Adults that harboured mutations caused by TALENs are underlined, while arrowheads indicate cleavage products from Surveyor nuclease assays. Arrows indicate 200-bp size marker. ( e – g ) Phenotypes of G 2 heterozygous and homozygous Gb ′ lac2 mutants generated with TALENs 1 day after hatching. Control first-instar nymphs were coloured black, while heterozygous mutants were still grey in colour and homozygous mutants were white. ( h ) Sequence analysis of Gb ′ lac2 mutant alleles induced by TALENs. The wild-type (WT) sequence is shown above the mutant sequences containing deletions (indicated with dashes) and/or insertions (shown in red letters). Boxed sequences represent TALEN-binding sites. Full size image Homozygous Gb ′ lac2 knockout nymphs generated using TALENs died in the first-instar stage, similar to knockout nymphs generated using ZFNs. When TALEN-induced Gb ′ lac2 mutants were crossed with ZFN-induced mutants, the resulting ZFN/TALEN homozygous Gb ′ lac2 knockout nymphs exhibited the same lethal effect as ZFN/ZFN knockout nymphs. These results indicate that the lethality observed is specific for the Gb ′ lac2 mutation, and is not due to mutations elsewhere in the genome. Moreover, we hypothesize that secondary consequences as a result of defects in the structural integrity of the cuticle in the absence of tanning are responsible for the lethality observed for homozygote crickets. Here an efficient approach for targeted mutagenesis and generation of biallelic (homozygous) knockouts in G. bimaculatus is reported. ZFNs and TALENs were used to induce germline mutations of exogenous and endogenous genes in the cricket genome. Via mutant screening steps using the Surveyor nuclease, we have successfully generated homozygous mutant crickets, which exhibit the knockout phenotype of the target gene, Gb ′ lac2 . This is the first research in hemimetabolous insects to show effectiveness of ZFNs and TALENs, and their capacity to generate knockout animals. Thus, an important advance in the ability to directly manipulate the genome of a non-traditional animal model is described, and it only requires the microinjection of ZFN/TALEN mRNAs and the identification of mutants using a Surveyor nuclease assay. In this study, a marker gene with a clear epidermal defect phenotype was used. However, the approach presented in this paper is able to generate knockout animals independent of a specific genotype or phenotype. Accordingly, this method represents a practical, and generally accessible, technique by which to affect any locus in the cricket genome, or any other genome, given that delivery of mRNA can be successful. The ZFN mRNA injection experiments performed resulted in 47–48% of fertile adults yielding mutant offspring. Combined with the sufficiently high frequency of NHEJ in crickets, it appears that our method can be used for: functional genomics in this species, disrupting specific coding sequences, and for targeting regulatory elements in the genome. In addition, the efficiency of generating founder animals using ZFNs is significantly higher than that observed for Bombyx mori [13] , and is comparable to that of Drosophila melanogaster ( Table 2 ) [11] . The disparity that exists between these species may be due to differences in the efficiency of mRNA incorporation into germline cells, and this may further depend on the mode of germ cell differentiation involved. In addition, differences in the binding affinity of ZFNs to target sequences may affect the efficiency of mutagenesis, especially as methods for ZFN design and screening differ between species. Following the injection of ZFN mRNAs into embryos, dose-dependent toxicity was found to be significantly higher for Gb ′ lac2 -targeted ZFNs than eGFP -targeted ZFNs. For example, lower concentrations of Gb ′ lac2 ZFN mRNA yielded decreased rates of early embryonic lethality and malformation. These results are consistent with those previously reported for Drosophila [10] , [32] , and suggest that dosage optimization for individual ZFN pairs is important for targeted mutagenesis, particularly to avoid unwanted genomic cleavage events. However, the target specificity demonstrated for Gb ′ lac2 -targeted ZFNs injected at 1 ng μl −1 indicates that specificity is sufficiently high, and no evidence of unwanted cleavage events were detected at nine other sites considered likely off-target genomic sites in Gb ′ lac2 knockout crickets. While these data do not rule out the possibility that off-target ZFN cleavage events occurred at other loci, the specificity profile obtained is promising. An advantage of using TALENs for genome editing is the greater flexibility in selecting target sequences versus ZFNs [33] . Our study is the first to demonstrate the capacity for TALENs to induce mutagenesis in insects other than Drosophila [24] . The rate of fertile adults that yielded mutant offspring in the present study (17%) also indicates that this method is suitable for practical use for cricket genome editing as well as ZFN-based mutagenesis. The frequency of NHEJ achieved in crickets used for TALEN experiments was lower than that of ZFN experiments performed for the same gene. However, mutation frequencies were not able to be directly compared between these experiments due to differences in the Fok I nuclease domains used (for example, heterodimer variants were used for ZFNs, and wild-type Fok I domains were used for TALENs). In addition, the targeted sequences were also different. In another report, engineered TALENs showed largely varying efficiencies of mutagenesis among 48 targeted sites in a single gene, or among 96 targeted genes in a human cell line [34] . Thus, it may be possible to achieve a higher efficiency of gene disruption using TALENs targeted to different sites. Unlike RNAi-based technologies, ZFN/TALEN-based technologies are able to generate gene knockouts and gene knock-ins. In addition, the possibility of off-targeting effects can be more rigorously excluded by checking potential target sequences in the genome. However, preparation of custom double-stranded RNAs is generally easier than generating custom ZFNs/TALENs, and accessibility to phenotypes is another advantage of RNAi. For example, following the injection of double-stranded RNA into eggs, phenotypes can be observed within a few days, rather than waiting for the next generation. The systemic effect of RNAi also enables the observation of phenotypes at a specific developmental stage, or in a specific organ, as previously demonstrated in the cricket with nymphal or regeneration-dependent RNAi experiments [25] , [26] , [27] . Thus, if used in combination, both ZFN/TALEN-based genome editing and RNAi-based targeting have the potential to greatly promote functional genomics. For example, in the cricket where RNAi-based functional screening has rapidly identified candidate genes involved in many biological processes (for example, leg regeneration, early embryogenesis [25] and memory formation [35] ), genome editing technologies can now be used to facilitate more detailed analyses of such genes using gene knock-out studies and the knock-in of reporter genes to obtain expression profiles. While there are many beneficial and deleterious species of insects, the latter is associated with an enormous amount of agricultural loss or fatal human disease. Currently, the well-established model insect systems that have been subject to sophisticated methods of genetic analysis and fully sequenced genomes (for example, fruitflies, red flour beetles and silkworms) are exclusively holometabolous (complete metamorphosis) species. However, many hemimetabolous species of insects (for example, aphids, cockroaches, crickets, grasshoppers) are significant agricultural pests or disease vectors. ZFNs/TALENs can be applied to the modification of genes responsible for deleterious traits in these insects, for example, to disrupt genes that facilitate the transmittal of pathogens, or to edit cis -regulatory regions of genes. Thus, the ability to edit the genomes of hemimetabolous insects using ZFNs/TALENs would facilitate the identification of new ways to address challenges posed by these insects, while avoiding the use of transgenic methods. This is in addition to contributing to genetic manipulation-based studies in other biological fields. Animals All adult and nymph two-spotted crickets, G. bimaculatus, were reared in plastic cases at 26–30 °C under a 10-h light, 14-h dark photoperiod. They were fed on artificial fish foods. For microinjections, fertilized eggs were collected on a wet kitchen towel and incubated at 28 °C in a plastic dish. Design and screening of ZFNs For designing ZFNs, the target sites of eGFP and Gb ′ lac2 genes were scanned for positions where 6 bp lies between 5′-NNC-3′ and 5′-GNN-3′ triplets. The ZF proteins generated included three ZF domains, with each domain capable of recognizing 3 bp of DNA. Target site selection also included the requirement that sequences with single-nucleotide polymorphisms were excluded, as Surveyor nuclease assays would be able to detect single-nucleotide polymorphisms as well as ZFN- or TALEN-induced mutations. Gb ′ lac2 ZFNs were designed to cleave a region encoding the catalytic domain of the Gb ′ lac2 gene. To screen for functional ZFNs, a bacterial one-hybrid system was used in combination with an SSA assay as described previously [17] . Briefly, randomized libraries of ZFs, containing fusion proteins of three-finger ZF arrays and the omega subunit of RNA polymerase, were co-transfected with HIS3 reporter vectors, containing the target sequences for ZF arrays, into the bacterial strain, US0D hisBDpyrFDrpoZ. Transfected bacteria were then plated on histidine-deficient plates with the HIS3 inhibitor, 3-amino-1,2,4-triazole. In SSA assays, a ZFN construct and a reporter construct containing a luciferase gene split into two inactive fragments by insertion of a stop codon and a pair of target sites were co-transfected into cultured cells. When a DSB at the target site is induced by a ZFN homodimer, SSA occurs between the homologous regions of the inactive fragments, thereby producing an active luciferase gene. eGFP ZFNs were assembled using DD/RR Fok I heterodimer variants, while Gb ′ lac2 ZFNs were assembled using DS/RR heterodimer sharky variants [29] , [31] . The design, construction and validation of TALENs targeting the Gb ′ lac2 gene ( Gb ′ lac2 TALENs L and R) were performed by Cellectis Bioresearch (Paris, France). Each TALEN recognized a 17-bp target site, and these sites were 23 bp apart. mRNA synthesis and microinjections into Gryllus eggs In vitro transcription of capped mRNA was performed using an mMESSAGE mMACHINE kit (Ambion, Austin, TX, USA) according to the manufacturer's instructions. Following ethanol precipitation, mRNAs were suspended in an appropriate volume of water to achieve a final concentration of 1 μg μl −1 for eGFP ZFNs and Gb ′ lac2 TALENs and 1 ng μl −1 for Gb ′ lac2 ZFNs. To perform microinjections of mRNA, cricket eggs were collected within 1 h of being laid and were used within 4 h of collection. The eggs were lined up on double-sided adhesive tape attached to a microscope slide after treatment with 70% ethanol for 10 s and wash. Solution containing mRNA was backloaded into a glass needle and injected into each egg at 20% in the egg length [26] . Analysis of mutations using Surveyor nucleases Primer pairs amplified a region of 400 and 210 bp containing the eGFP and Gb ′ lac2 target sites, respectively. To detect eGFP - or Gb ′ lac2 -ZFN-induced mutations in G 0 embryos, we extracted genomic DNA of 25 embryos at 7 or 2 days after injection, respectively, and used them for the Surveyor nuclease assays. For the first round of screening in the ZFN/TALEN experiments, genomic DNA of 25 G 1 embryos at 7 days after egg laying were used in each line. For the second round of Surveyor nuclease assays, genomic DNA was extracted from T3 legs of G 1 final-instar nymphs. To allow complementary but mismatched strands to anneal, PCR products (10 μl) were incubated at 95 °C for 5 min, 95 °C for 85 °C at −2 °C s −1 and 85 °C to 25 °C at −0.1 °C s −1 . Nuclease S (0.5 μl) and Enhancer S (0.5 μl) (Surveyor Mutation Detection Kit, Transgenomic, Omaha, NE, USA) were then added and samples were incubated at 42 °C for 20 min to digest the annealed PCR products at the sites of mismatch. Nuclease S-digested PCR products were analysed by agarose gel electrophoresis. How to cite this article: Watanabe, T. et al . Non-transgenic genome modifications in a hemimetabolous insect using zinc-finger and TAL effector nucleases. Nat. Commun. 3:1017 doi: 10.1038/ncomms2020 (2012).